A toxin-antidote system contributes to interspecific reproductive isolation in rice Breakdown of reproductive isolation facilitates flow of useful trait genes into crop plants from their wild relatives. Hybrid sterility, a major form of reproductive isolation exists between cultivated rice ( Oryza sativa ) and wild rice ( O. meridionalis , Mer ). Here, we report the cloning of qHMS1 , a quantitative trait locus controlling hybrid male sterility between these two species. Like qHMS7 , another locus we cloned previously, qHMS1 encodes a toxin-antidote system, but differs in the encoded proteins, their evolutionary origin, and action time point during pollen development. In plants heterozygous at qHMS1 , ~ 50% of pollens carrying qHMS1- D (an allele from cultivated rice) are selectively killed. In plants heterozygous at both qHMS1 and qHMS7, ~ 75% pollens without co-presence of qHMS1-Mer and qHMS7- D are selectively killed, indicating that the antidotes function in a toxin-dependent manner. Our results indicate that different toxin-antidote systems provide stacked reproductive isolation for maintaining species identity and shed light on breakdown of hybrid male sterility. Reproductive isolation is a common phenomenon in nature and exists in different forms. Depending on species, reproductive barriers can occur either before (pre-zygotic) or after (post-zygotic) fertilization. In plants, the pre-zygotic barriers include geographical isolation, differentiations in flower habit, failure in cell-to-cell recognition between the pollen and stigma, inability in pollen germination and pollen tube growth, and defects in cell fusion between sexual gametes. For example, the speciation locus YUP in mokeyflowers [1] , the unilaterally incompatibility system found in Brassicaceae [2] , [3] , Zea mays [4] , [5] , [6] , [7] and tomato [8] , [9] , [10] is the well-studied pre-zygotic mechanism. Post-zygotic reproductive isolation (also called hybrid incompatibility) has been extensively studied in animals, plants and microorganisms that include hybrid sterility (HS) and hybrid necrosis or weakness. HS is a common hybrid incompatibility. The toxin-antidote system (sometimes called killer-protector, meiotic drive, gene drive and segregation distortion in different literatures) is one of the genetic mechanisms conferring HS in animals and plants [11] . Genetic elements belonging to this group include the segregation distorter ( SD) system in Drosophila [12] , [13] , the wtf loci in yeast [14] , [15] , the peel-1/zeel-1 and sup35/pha-1 genes in nematodes [16] , [17] , [18] , the t -haplotype in mice [19] , [20] , [21] , the Spok [22] and het-s genes [23] in Podospora anserina , the Sk genes in Neurospora [24] , and APOK3 in Arabidopsis [25] . In those systems the cells/gametes that do not contain a functional antidote are selectively killed. Thus, the toxin-antidote systems evolved during speciation likely play a key role to maintain species identity. Although also being common in plants, only one HS case in Arabidopsis and a few in rice have been deciphered to causal genes. The Arabidopsis APOK3 encodes an antidote, functioning according to the toxin-antidote model to destroy the pollen-killer activity conferred by three genetically linked elements [25] . In rice, the S27/S28 [26] , DPL1/DPL2 [27] and DGS1/DGS2 [28] are pairs of duplicated genes, and pollens carrying malfunctioned alleles at both of the paired loci are defective in development, leading to HS in hybrid plants. The genes encoding those systems are usually located in separated loci and how they evolved during speciation has been hypothesized in the Bateson-Dobzhansky-Muller model [29] , [30] . Sometimes, the toxin-antidote (or killer-protector) genes are tightly linked at a single locus, including the male HS loci qHMS7 [31] , Sa [32] , the female HS locus S5 [33] and the female-male HS locus S1 [34] , [35] , [36] . In heterozygotes, those gametes carrying non-functional antidote or protector genes are unable to develop to maturity. In a special case, the two alleles of the Sc locus encode homologs of DUF1618 domain protein that is essential for pollen development but are different in copy number and promoter region [37] . In F 1 hybrids ( Sc-j/Sc-i ), Sc-i (more copies) is expressed whereas Sc-j (single copy) is suppressed, such that the pollens carrying Sc-i are selectively transmitted. How those genes at a single locus have been co-evolved remains elusive. Of those cloned rice systems, only qHMS7 was based on HS between wild and cultivated rice, and all the others on HS between subspecies of O. sativa or between the two cultivated species O . sativa and O . glaberrima (the S1 locus). Therefore, more efforts need to be put into uncovering genetic mechanisms underlying interspecific HS between wild and cultivated rice. There are eight Oryza species in the AA genome group, including the two cultivated rice species and O. meridionalis ( Mer ) from Australia that is considered the earliest divergent lineage around 2.93 mya [38] . We assume that cloning and characterization of reproductive isolation genes between cultivated rice and Mer would provide not only their evolutionary trajectory but also strategic designs to break reproductive isolation and bridge gene flow from other wild relatives downstream of Mer to cultivated rice. To this end, we constructed mapping populations derived from the cross between Mer and Dianjingyou 1 (DJY1), a japonica subspecies cultivar of O. sativa . The F 1 hybrid plants of DJY1 and Mer are completely male-sterile and four underlying major quantitative hybrid male sterility loci ( qHMS1 , qHMS2 , qHMS7 and qHMS9 , located on chromosome 1, 2, 7, and 9, respectively) were detected [31] . Among those, qHMS7 has been cloned and shown to encode a toxin-antidote element and kill pollens carrying the Mer allele [31] . The genetic mechanisms of other three loci are still unknown. In this study, we construct a near isogenic line NIL- qHMS1 in DJY1 background but contains the qHMS1 locus from Mer , and clone qHMS1 . The Mer allele of qHMS1 encodes a functional toxin-antidote system and kills pollens carrying the non-functional DJY1 allele. The breakdown of the qHMS1 locus is a recent event as it is only found in Asian cultivated rice species and their closest wild progenitors. When qHMS1 is stacked with qHMS7 in the DJY1 background, majority of pollens (~75%) in heterozygotes are aborted. This reconstructed HS mimics reproductive isolation and provides insights into how the stacked HS genetic systems contribute to maintaining species identity. Mer allele of qHMS1 causes development defect in pollens carrying DJY1 allele To clone qHMS1 , we developed a near-isogenic line (NIL) harboring the Mer allele of qHMS1 in the DJY1 background (designated NIL- qHMS1 ) (Supplementary Fig. 1 ). NIL- qHMS1 was morphologically similar to DJY1 and produced fertile pollens, but their hybrid F 1 plants (DJY1/NIL- qHMS1 ) produced ~50% aborted pollens (Fig. 1a–d , Supplementary Fig. 2 ). Examination of a BC 5 F 2 population revealed a clear-cut bimodal distribution in pollen fertility (Supplementary Fig. 3 ). Further genotyping analysis of this population with molecular markers revealed that individuals homozygous for the Mer allele and those heterozygotes carrying both Mer and DJY1 alleles segregated at a 1:1 ratio, with very few plants (1.1%) homozygous for the DJY1 allele, suggesting that the Mer allele was selectively transmitted to progeny (Fig. 1e ). Moreover, a reciprocal cross test between DJY1 and F 1 (DJY1/NIL- qHMS1 ) resulted in only heterozygous progeny when DJY1 was used as the female parent and ~50% DJY1/DJY1 progeny when F 1 was used as the female (Fig. 1f ). In addition, the average seed setting rate of the BC 5 F 2 population was >85%, indicating normal spikelet fertility regardless of genotypes (Supplementary Fig. 4 ). These results collectively demonstrate that the qHMS1 locus from Mer encodes a selfish genetic element and controls hybrid sterility by eliminating male gametes carrying the counterpart from cultivated rice. Fig. 1: Cloning of the qHMS1 locus underlying the semi-sterile pollen phenotype. a – c Normal fertile pollens in DJY1 ( a ) and NIL- qHMS1 ( c ) and aborted pollens in their F 1 plant ( b ), as shown by I 2 -KI staining to indicate starch accumulation. Scale bar, 100 μm. d Quantification of pollen fertility in DJY1, NIL- qHMS1 and their F 1 shown as means ± SD ( n = 10 plants). The semi-sterile pollen phenotype was seen in F 1 . **P = 3.47752E-9 < 0.01 by two-tailed student’s t test; NS, no significance. e Genotypic distribution at qHMS1 among a BC 5 F 2 population. Few plants were found homozygous for the D allele, verifying the failure of its transmission through pollen. D , DJY1 allele; M , Mer allele. f Selective transmission of the Mer allele through pollen as tested in reciprocal crosses between DJY1 and F 1 (DJY1/NIL- qHMS1 ). Plants derived from the crosses were genotyped using molecular markers to distinguish origin of the qHMS1 alleles. g qHMS1 was anchored to a 43-kb region on chromosome 1. Numbers under the black bar indicate recombinants between markers. FF, fully fertile; SS, semi-sterile; F 2:3 , progeny of selected F 2 recombinants. Pollen fertility of these recombinants shown as means ± SD ( n = 3 indepe n dent spikelets). h Genomic structure of the two candidate genes constituting a selfish genetic element. Vertical bars indicate exons. Position of single nucleotide polymorphisms (SNP) and transposon insertion is shown relative to the start codon. The two SNPs in the coding regions are highlighted in blue. TE, transposable element. Two black triangles indicate a 19-bp and a 235-bp insertion, respectively. Source data are provided as a Source Data file. Full size image Histochemical investigation revealed that there was no developmental defect seen from meiosis until the early uninucleate stage in DJY1/NIL- qHMS1 F 1 anthers (Supplementary Fig. 5 ). After that, however, diffused nucleus appeared in part of microspores that did not undergo first mitosis and finally developed to hollow pollens lacking nuclei and without starch accumulation (Supplementary Figs. 6 , 7 ), although the surface and wall structure of the aborted pollens were similar to normal pollens (Supplementary Fig. 8 ). Thus, the pollen abortion is likely attributed to the failure of first mitosis during the gametophytic development. Cloning and genomic structure of qHMS1 To clone qHMS1 , we first used 356 BC 5 F 2 plants and mapped qHMS1 to a region flanked by the molecular makers CH1-11 and RM3475 on chromosome 1. Using 11,800 BC 5 F 3 progeny derived from BC 5 F 2 plants heterozygous at qHMS1 , we further narrowed down the locus to a 43-kb region, which was subsequently confirmed by examination of the recombinant offspring (Fig. 1g ). Based on the annotation of the O. sativa Japonica Group IRGSP-1.0 ( http://www.gramene.org/ ), this region is predicted to contain five open reading frames ( ORF s) (Fig. 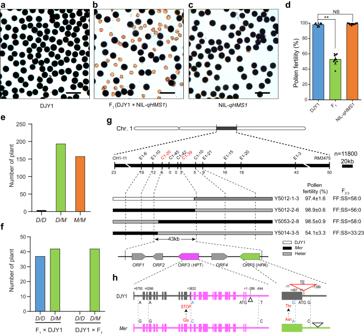Fig. 1: Cloning of theqHMS1locus underlying the semi-sterile pollen phenotype. a–cNormal fertile pollens in DJY1 (a) and NIL-qHMS1(c) and aborted pollens in their F1plant (b), as shown by I2-KI staining to indicate starch accumulation. Scale bar, 100 μm.dQuantification of pollen fertility in DJY1, NIL-qHMS1and their F1shown as means ± SD (n= 10 plants). The semi-sterile pollen phenotype was seen in F1.**P= 3.47752E-9 < 0.01 by two-tailed student’sttest; NS, no significance.eGenotypic distribution atqHMS1among a BC5F2population. Few plants were found homozygous for theDallele, verifying the failure of its transmission through pollen.D, DJY1 allele;M,Merallele.fSelective transmission of theMerallele through pollen as tested in reciprocal crosses between DJY1 and F1(DJY1/NIL-qHMS1). Plants derived from the crosses were genotyped using molecular markers to distinguish origin of theqHMS1alleles.gqHMS1was anchored to a 43-kb region on chromosome 1. Numbers under the black bar indicate recombinants between markers. FF, fully fertile; SS, semi-sterile; F2:3, progeny of selected F2recombinants. Pollen fertility of these recombinants shown as means ± SD (n= 3 independent spikelets).hGenomic structure of the two candidate genes constituting a selfish genetic element. Vertical bars indicate exons. Position of single nucleotide polymorphisms (SNP) and transposon insertion is shown relative to the start codon. The two SNPs in the coding regions are highlighted in blue. TE, transposable element. Two black triangles indicate a 19-bp and a 235-bp insertion, respectively. Source data are provided as a Source Data file. 1h , Supplementary Table 1 ). Sequence comparison between Mer and DJY1 revealed no difference in ORF1 , a single base change in ORF2 , and a 615-bp deletion and five SNPs in ORF4 (Supplementary Fig. 9a ). In DJY1 ORF3 , a single base change from G to T was found, leading to an early stop codon (Fig. 1h ). In DJY1 ORF5 , a T-to-C base substitution results in an amino acid change of Asn to Thr, in addition to a 1391-bp transposon inserted 11-bp upstream of the ATG start codon (Fig. 1h ). Then RNA sequencing (RNA-seq) experiment was performed to analyze the expression of genes in the mapping region and the results showed that ORF1-ORF3 and ORF5 , but not ORF4 , are expressed in developing anther (Supplementary Fig. 9b ). ORF3/HPT encodes a toxin protein To further dissect the qHMS1 locus, we performed targeted mutagenesis to all the five genes using the CRISPR-Cas9 technology. Loss-of-function mutation of ORF1 , ORF2 and ORF4 in DJY1/NIL- qHMS1 F 1 plants did not change the semi-sterile phenotype, thus excluding their role in male sterility control (Supplementary Fig. 10 ). Then we focused on ORF3 first and produced ORF3 knock-out lines in the DJY1/NIL- qHMS1 F 1 background using the CRISPR-Cas9 technology. We investigated three lines each representing a unique editing type in T 0 or T 1 plants and found that loss-of-function mutation of ORF3 rescued pollen fertility (Fig. 2a–f ). As expected, the segregation of three genotypes at qHMS1 fits into the 1:2:1 ratio in the self-bred offspring of the knockout lines and the DJY1 allele of qHMS1 was transmitted to progeny (Fig. 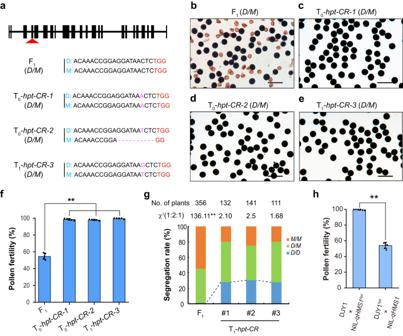Fig. 2:HPTfunctions as a toxin. aCreation of edited F1(DJY1/NIL-qHMS1) plants. The target site is indicated by red arrowhead. The PAM (TGG) is highlighted by red, and inserted bases by pink and deletion by pink dotted line. Two primary (T0) and one progeny (T1) plants are presented.b–ePollen semi-sterility in transgene-negative F1(b) and restored pollen fertility in edited T0(c,d) and T1(e) plants. Scale bar, 100 μm.fQuantification of pollen fertility in plants shown in (a). Data are means ± SD (n= 5 independent spikelets).**P= 1.60116E-5 < 0.01 by two-tailed student’sttest.gSegregation of genotypes atqHMS1fits into the 1:2:1 ratio upon knocking-out ofHPT.**P≈ 0 < 0.01 in χ² test.hVerification ofHPTfromMeras a functional toxin.HPTwas knocked out in DJY1 (DJY1hpt) or NIL-qHMS1(NIL-qHMS1hpt)background and F1was made by crossing for pollen fertility test. Data are means ± SD (n= 6 plants).**P= 9.26256E-10 < 0.01 by two-tailed student’sttest. Source data are provided as a Source Data file. 2g , Supplementary Table 2 ). Moreover, introduction of a genomic fragment harboring ORF3 from Mer into DJY1 resulted in full pollen sterility, whereas knocking-out of ORF3 in DJYI (DJY1 orf3 ) or NIL- qHMS1 (NIL- qHMS1 orf3 ) showed no impact on pollen fertility as well as plant growth and development, indicating its exclusive role as a toxin (Supplementary Fig. 11 ). Further, F 1 plants from the cross of DJY1 orf3 with NIL- qHMS1 were still semi-sterile whereas those F 1 plants from the cross of DJY1 with NIL- qHMS1 orf3 were fully fertile, confirming that it is the ORF3 from Mer that encodes a functional toxin (Fig. 2h ). We thus named the gene as HPT ( Hybrid Pollen Toxin ) hereafter. Fig. 2: HPT functions as a toxin. a Creation of edited F 1 (DJY1/ NIL-qHMS1 ) plants. The target site is indicated by red arrowhead. The PAM (TGG) is highlighted by red, and inserted bases by pink and deletion by pink dotted line. Two primary (T 0 ) and one progeny (T 1 ) plants are presented. b – e Pollen semi-sterility in transgene-negative F 1 ( b ) and restored pollen fertility in edited T 0 ( c , d ) and T 1 ( e ) plants. Scale bar, 100 μm. f Quantification of pollen fertility in plants shown in ( a ). Data are means ± SD ( n = 5 independent spikelets). **P = 1.60116E-5 < 0.01 by two-tailed student’s t test. g Segregation of genotypes at qHMS1 fits into the 1:2:1 ratio upon knocking-out of HPT . **P ≈ 0 < 0.01 in χ² test. h Verification of HPT from Mer as a functional toxin. HPT was knocked out in DJY1 (DJY1 hpt ) or NIL- qHMS1 (NIL- qHMS1 hpt ) background and F 1 was made by crossing for pollen fertility test. Data are means ± SD ( n = 6 plants). **P = 9.26256E-10 < 0.01 by two-tailed student’s t test. Source data are provided as a Source Data file. Full size image ORF5/HPA encodes an antidote protein The fact that HPT is not toxic to its host pollen infers that the Mer allele of qHMS1 may harbor an antidote element. Accordingly, we focused on the remaining gene ORF5 contained in the mapped region. We also used the CRISPR-Cas9 technology to produce loss-of-function mutation of ORF5 in the same DJY1/NIL- qHMS1 F 1 background and found that the knock-out line showed complete sterility, instead of ~50% male sterility (Fig. 3b, e ). Subsequently, we knocked out ORF5 in both DJY1 (homozygous for the ORF5 -D allele and fully fertile) and NIL- qHMS1 (homozygous for the ORF5 - Mer allele and fully fertile) and found that the DJY1 orf5 plant was still fully fertile but the NIL- qHMS1 orf5 plant lost pollen fertility completely (Fig. 3a–d ). Those results indicate that ORF5 encodes an antidote detoxifying the toxin protein HPT of the Mer origin and that only the one from Mer is functional. We thus named ORF5 as HPA ( Hybrid Pollen Antidote ) hereafter. This notion was supported by introduction of a Mer genetic fragment containing intact HPA into DJY1/NIL- qHMS1 F 1 , which restored male fertility from ~50% to ~75% in single-copy transgenic plants (Fig. 3f–h ). Genotyping of the progeny showed that all the offspring homozygous for the DJY1 allele of qHMS1 carried the HPA transgene, suggesting the cis -acting nature of HPA (Fig. 3i , Supplementary Tables 3 , 4 ). Collectively, those results indicate that HPT and HPA from Mer together constitute a selfish genetic element. Fig. 3: HPA functions as an antidote. a Target site in HPA (top) for CRISPR/Cas9-mediated mutagenesis and a HPA genomic fragment from Mer (bottom) for genetic complementation test. PAM is highlighted in red. b Pollen fertility in knock-out ( hpa-CR ) and complementation ( gHPA-COM ) lines. Data are means ± SD ( n = 5 independent spikelets). **P = 1.21003E-10 of NIL- qHMS1 vs hpa-CR-1 , 2.27263E-5 of F 1 vs hpa-CR-2 , 0.00075 of F 1 vs gHPA-COMs < 0.01 by two-tailed student’s t test. c – h Representative images of pollen phenotype in wild type (WT) ( c ) and knock-out ( d ) of NIL- qHMS1 , and knock-out ( e ), WT ( f ) and complemented ( g , h ) lines of F 1 (DJY1/ NIL- qHMS1 ). Scale bar, 100 μm. i Observed segregation rate among progeny of the complemented lines, showing successful transmission of the DJY1 allele of qHMS1 . **P = 9.613E-7 < 0.01 in χ² test. Source data are provided as a Source Data file. Full size image Truncation of HPT and a transposon insertion in HPA leads to the non-functional DJY1 allele HPT encodes a member of the helicase subfamily, containing two RRM (RNA recognition motif) domains located in the N terminal, a DEAD-like helicases c domain (DEXDc), a Helicase superfamily c-terminal (HELICc) domain and a coiled coil (CC). The single base change of G to T in DJY1 leads to an early stop codon, truncating HPT from 902 amino acids (aa) to 670 aa, with both the HELICc and CC domains removed (Fig. 1h , Supplementary Fig. 12a ). RNA-seq analysis of anthers at S9-S11 (early microspore stage (S9), vacuolated microspore stage (S10) and bicellular stage (S11)) revealed similar read depths between NIL- qHMS1 , DJY1 and their F 1 plants across HPT (Supplementary Fig. 13a ). HPT transcript was detectable in all the sampled tissues collected from plants at the flowering stage, with the preferred expression in the anther; and further analysis in developing anthers showed higher expression of HPT starting from early uninucleate stage (S9) through maturation of the pollen (S13) (Supplementary Fig. 13b, c ). The HPT promoter regions from Mer and DJY1 have similar activity as shown using the luciferase (LUC) reporter gene (Supplementary Fig. 13d ). HPT was localized in both nucleus and cytoplasm in the transient protoplast assays and the truncated version from DJY1 retains its subcellular localization (Supplementary Fig. 14 ). Those results suggest that it is the truncation event that destroys toxicity of HPT in DJY1. The requirement of the C-terminal for functioning of HPT, where the HELICc and CC domains reside, was verified with a non-functional HPT created by a frameshift mutation near the G-to-T mutation in DJY1/NIL- qHMS1 F 1 (Supplementary Fig. 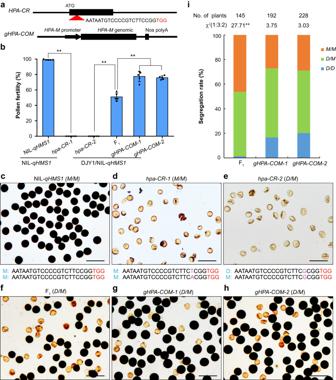Fig. 3:HPAfunctions as an antidote. aTarget site inHPA(top) for CRISPR/Cas9-mediated mutagenesis and aHPAgenomic fragment fromMer(bottom) for genetic complementation test. PAM is highlighted in red.bPollen fertility in knock-out (hpa-CR) and complementation (gHPA-COM) lines. Data are means ± SD (n= 5 independent spikelets).**P= 1.21003E-10 of NIL-qHMS1vshpa-CR-1, 2.27263E-5 of F1vshpa-CR-2, 0.00075 of F1vsgHPA-COMs< 0.01 by two-tailed student’sttest.c–hRepresentative images of pollen phenotype in wild type (WT) (c) and knock-out (d) of NIL-qHMS1, and knock-out (e), WT (f) and complemented (g,h) lines of F1(DJY1/ NIL-qHMS1). Scale bar, 100 μm.iObserved segregation rate among progeny of the complemented lines, showing successful transmission of the DJY1 allele ofqHMS1.**P= 9.613E-7 < 0.01 in χ² test. Source data are provided as a Source Data file. 15 ). HPA encodes an F-Box protein of 361 aa, with the F-Box motif located at the N-terminal, having two exons in its genomic structure (Fig. 1h , Supplementary Fig. 12b ). Profiling of Mer HPA expression in the NIL- qHMS1 background indicates much preferred transcript accumulation in anthers, which reaches a peak at anther development stages S9-S10, roughly equivalent to early and late uninucleate pollens, respectively (Supplementary Fig. 13e, f ). The anther-preferred expression of HPA was verified using the GUS reporter gene driven by a 1.4-kb promoter fragment of Mer -type HPA (Supplementary Fig. 13g ). HPA was exclusively localized in nucleus (Supplementary Fig. 14 ). Next we investigated whether the 1391-bp transposon inserted 11-bp upstream of the ATG start codon or the single base change of T to C (Asn to Thr at aa level), or both, impact on the function of HPA at the DJY1 allele (Fig. 1h ). We performed RNA-seq analysis on anthers of NIL- qHMS1 , DJY1 and their F 1 , and found no transcript reads corresponding to the HPA coding region only in DJY1, implying that the transposon insertion disrupts transcription of HPA (Fig. 4a ). The insertion-associated promoter inactivation was verified in the protoplast transient assay using LUC as a reporter (Fig. 4b ). Further, RNA in situ hybridization on floral sections detected signal in NIL- qHMS1 but not or faint signal in DJY1 (Supplementary Fig. 16 ). The promoter swapping experiment between DJY1 and Mer confirmed functionality of the DJY1-type HPA coding sequence, regardless of the Asn to Thr Amino acid substitution (Fig. 4c–e ). Thus, it is the transposon insertion rather than the single base substitution that leads to no accumulation of the antidote in pollens carrying the DJY1 allele of qHMS1 . Fig. 4: A transposon insertion in HPA promoter region inactivates its transcriptional activity. a RNA-seq analysis did not detect transcription from the coding region of HPA in DJY1 whereas HPA was transcribed in NIL- qHMS1 and their F 1 . TE region, transposon insertion region. 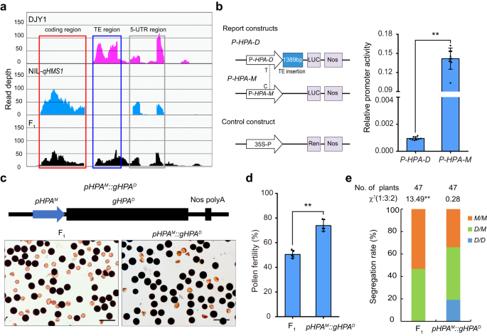Fig. 4: A transposon insertion inHPApromoter region inactivates its transcriptional activity. aRNA-seq analysis did not detect transcription from the coding region ofHPAin DJY1 whereasHPAwas transcribed in NIL-qHMS1and their F1. TE region, transposon insertion region.bPromoter activity comparison ofHPAbetween DJY1 andMer. The promoter region from DJY1 (P-HPA-D, containing the transposon) orMer(P-HPA-M) were used to drive the firefly luciferase (LUC) reporter gene in the protoplast transient assay. The Renilla luciferase gene driven by 35 S promoter was used as an internal control for data normalization. Data are means ± SD (n= 9 biologically independent samples).**P= 6.10922E-09 < 0.01 by two-tailed student’sttest.cThe detoxification role ofHPAfrom DJY1 is restored upon being transcribed. The DJY1HPApromoter was replaced with the one fromMerand the resulting vector (pHPAM::gHPAD) was transformed into F1(DJY1/NIL-qHMS1). Representative images show partial restoration of pollen fertility. Scale bar, 100 μm.dQuantification of pollen fertility inpHPAM::gHPADplants. Data are means ± SD (n= 4 independent spikelets).**P= 0.00053 < 0.01 by two-tailed student’sttest.eSegregation of genotypes atqHMS1among progeny of a single-copypHPAM::gHPADplant.**P= 0.001177 < 0.01 in χ² test. Source data are provided as a Source Data file. b Promoter activity comparison of HPA between DJY1 and Mer . The promoter region from DJY1 ( P-HPA-D , containing the transposon) or Mer ( P-HPA-M ) were used to drive the firefly luciferase (LUC) reporter gene in the protoplast transient assay. The Renilla luciferase gene driven by 35 S promoter was used as an internal control for data normalization. Data are means ± SD ( n = 9 biologically independent samples). **P = 6.10922E-09 < 0.01 by two-tailed student’s t test. c The detoxification role of HPA from DJY1 is restored upon being transcribed. The DJY1 HPA promoter was replaced with the one from Mer and the resulting vector ( pHPA M ::gHPA D ) was transformed into F 1 (DJY1/NIL- qHMS1 ). Representative images show partial restoration of pollen fertility. Scale bar, 100 μm. d Quantification of pollen fertility in pHPA M ::gHPA D plants. Data are means ± SD ( n = 4 independent spikelets). **P = 0.00053 < 0.01 by two-tailed student’s t test. e Segregation of genotypes at qHMS1 among progeny of a single-copy pHPA M ::gHPA D plant. **P = 0.001177 < 0.01 in χ² test. Source data are provided as a Source Data file. Full size image To detect whether HPA directly interacts with HPT, we performed yeast two-hybrid and in vitro pull-down assays. The results showed no physical interaction between these two proteins (Supplementary Fig. 17 ). Helicase subfamily genes have previously been reported to perform diverse cellular functions in virtually all steps of RNA metabolism from bacteria to humans. With this knowledge, we performed RNA-seq experiments on anthers from the gHPT-COM transgenic plant carrying the HPT - Mer genetic fragment and displaying full pollen sterility in the DJY1 background, and DJY1 as a control (Supplementary Fig. 18a, b ). The anthers were sampled at the meiotic stage (S8) and the uninucleate stage (S9-S10) at which the first mitosis was arrested (Supplementary Fig. 6 ). The results showed that there were 3520 differentially expressed genes (DEGs) at the meiotic stage, with 2103 down-regulated and 1417 up-regulated (Supplementary Fig. 18c ). Among the 2103 DEGs, 61 were down-regulated by 20 folds, of which 21 are anther-specific expressed (Supplementary Data 1 ; http://rapdb.dna.affrc.go.jp ). At the uninucleate stage, there were 4905 DEGs, with 2717 down-regulated and 2188 up-regulated (Supplementary Fig. 18d ). Among the 2717 DEGs, 20 were down-regulated by 20 folds, of which 7 are anther-specific expressed (Supplementary Data 1 ). Then we combined data from the two stages and identified 1953 co-DEGs, with 1243 down-regulated and 710 up-regulated (Supplementary Fig. 18e, f ). GO analysis on those 1243 genes indicated that they were clustered in various pathways and cellular processes, particularly in the processing and metabolism of ncRNA and rRNA (Supplementary Fig. 18g ). KEGG analysis on the same DEGs revealed various metabolic pathways, especially in the sugar and starch metabolisms (Supplementary Figs. 18 h, 19 ). We performed qRT-PCR on some of those glycolysis or gluconeogenesis-related DEGs and confirmed their down-regulated expression in the gHPT-COM transgenic plant (Supplementary Fig. 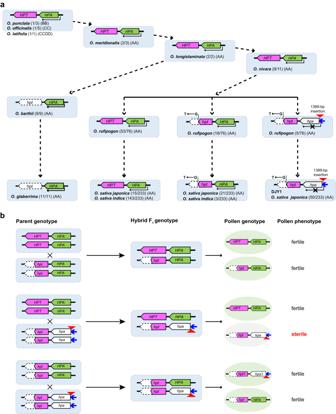Fig. 5: Loss-of-function ofqHMS1is a recent evolutionary event. aCoupling of the toxin HPT with the antidote HPA. Mutation ofHPTandHPAwas found in cultivated rice and its closest progenitor in Asia and Africa. Mutation ofHPAis conditioned by mutatedHPT. Loss or truncation of HPT is indicated by white bars with dotted line. Inactivation ofHPAtranscription due to the transposon insertion is indicated by white bars with black line. Shown in parenthesis is number of a given genotype over total accessions analyzed.bPredicted hybrid pollen sterility in combinations between the twoqHMS1alleles as a guide in breeding programs. The varieties with mutatedHPTbut functionalHPAare considered having wide compatibility. The combination that produces pollen sterility is highlighted in red rectangle. 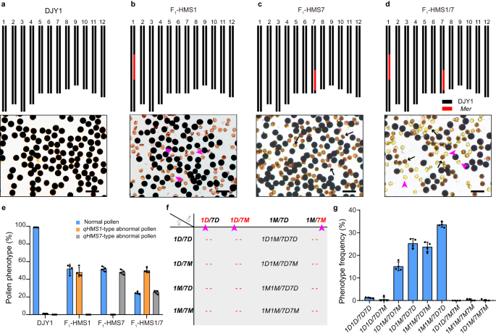Fig. 6:qHMS1andqHMS7are independent in action and together provide tiered hybrid male sterility. a–dChromosome location ofqHMS1andqHMS7and representative images of pollen phenotype in DJY1 (a), DJY1/qHMS1F1(F1-HMS1) (b), DJY1/qHMS7F1(F1-HMS7) (c) andqHMS1/qHMS7F1(F1-HMS1/7) (d). The pollen abortion caused byqHMS1at uninucleate stage and that caused byqHMS7at binucleate stage are indicated by pink arrowheads and black arrows, respectively. Scale bar, 100 μm.eQuantification of pollen phenotypes in hybrid plants. Data are means ± SD (n= 5 independent spikelets).fExpected genotypes among progeny of F1-HMS1/7. Pink arrowheads indicate the aborted pollen.1D, DJY1 allele ofqHMS1;1M,Merallele ofqHMS1;7D, DJY1 allele ofqHMS7;7M,Merallele ofqHMS7.gGenotypic distribution among progeny of F1-HMS1/7 plants (n= 4 F2populations from four randomly chosen F1plants). The prevalence of the four genotypes verifies the expectation inf. Note the uneven distribution frequency of the four genotypes. The female gametes carrying both the functional TAs (1 M/7D) have the highest transmission whereas those carrying both the none-functional TAs (1D/7 M) have the lowest transmission, suggesting that two TAs together can build up partial hybrid female sterility. Four F2populations (100–200 plants each) from 4 randomly chosen F1plants were genotyped. Data are means ± SD. Source data are provided as a Source Data file. 20 , Supplementary Table 5 ). Together, those results suggest a possible role of HPT in interfering expression of sugar/starch metabolic genes, which in turn may affect subsequent starch granule formation during pollen development, leading to final pollen abortion. qHMS1 has evolved non-functional alleles in cultivated rice and its closest wild relatives Using 100 wild rice and 244 landrace varieties (Supplementary Data 2 ), we traced the evolutionary trajectory of the HPT and HPA from Mer to cultivated rice. For HPT , the genomic sequence is identical in earlier wild species of the AA genomes group, but changes were found in O . barthii , the wild progenitor of cultivated rice in Africa, and in O . rufipogon , the wild progenitor of cultivated rice in Asia (Fig. 5a , Supplementary Fig. 21a ). HPT is lost in all the O . barthii accessions and cultivated African landraces ( O . glaberrima ) analyzed. HPT is diversified in O . rufipogon , with majority of accessions (53 out of 76) retaining the Mer version of HPT and minority (23 out of 76) having evolved the DJY1 version (with early stop due to the G to T mutation). In 233 descendants ( O . sativa ) of O . rufipogon , 67.8% landraces carry Mer HPT and 32.2% carry DJY1 HPT (Fig. 5a ). Thus, loss-of-function of HPT is a recent evolutionary event. The similar frequencies of Mer HPT and DJY1 HPT between O . rufipogon and O . sativa suggest that HPT was not selected during domestication of cultivated rice. Fig. 5: Loss-of-function of qHMS1 is a recent evolutionary event. a Coupling of the toxin HPT with the antidote HPA. Mutation of HPT and HPA was found in cultivated rice and its closest progenitor in Asia and Africa. Mutation of HPA is conditioned by mutated HPT . Loss or truncation of HPT is indicated by white bars with dotted line. Inactivation of HPA transcription due to the transposon insertion is indicated by white bars with black line. Shown in parenthesis is number of a given genotype over total accessions analyzed. b Predicted hybrid pollen sterility in combinations between the two qHMS1 alleles as a guide in breeding programs. The varieties with mutated HPT but functional HPA are considered having wide compatibility. The combination that produces pollen sterility is highlighted in red rectangle. Full size image For HPA , its protein coding region remains unchanged in all the analyzed accessions, including wild and cultivated rice, except the single T to C mutation that has no impact on function of HPA as described above (Fig. 4c–e ). The transposon insertion in the HPA promoter region exists in 6.6% (5/76) O . rufipogon (Supplementary Fig. 21b ) and 21.9% (51/233) O . sativa accessions, particularly only in some (51/87) of O . sativa ssp. japonica rice (Fig. 5a ). Interestingly, HPA remains intact in African rice where HPT no longer exists. It is likely that the insertion event occurred after the loss-of-function mutation of HPT as the site-specific insertion in HPA does not exist in the context of a functional HPT , or any loss-of-function mutation of HPA would not survive at the presence of Mer HPT (Fig. 5a ). The fact that the functional HPT must be coupled with the expressed HPA is also true in recently sequenced 251 and 33 varieties representing diverse genetic backgrounds [39] , [40] (Supplementary Data 2 ), which at least partially explains why the silenced HPA exists at a lower frequency. We constructed a phylogenetic tree based on HPA sequences in the eight rice species of the AA genome group. This tree shows again the co-evolution of silenced HPA with the non-functional allele of HPT (Supplementary Fig. 22 ). Accordingly, we propose a model that would provide a guide in choosing parents for hybrid breeding in consideration of pollen fertility (Fig. 5b ). An extended protein sequence analysis to more distant species, including wheat and sorghum, suggests possible conservation of these two proteins, particularly the F-Box in HPA and DEXD and HELICc domains in HPT (Supplementary Figs. 23 , 24 , Supplementary Tables 6 , 7 ). Whether those distant versions have function in maintaining species identity remains to be elucidated. qHMS1 provides the first tier of hybrid sterility in a genetic stack with qHMS7 The newly evolved functional DJY1 allele at the qHMS7 locus kills the pollen carrying the non-functional Mer allele [31] , opposite to the qHMS1 locus where the functional Mer allele kills the pollen carrying the newly evolved non-functional DJY1 allele as shown in this study. We therefore brought those two loci together by crossing NIL- qHMS1 with NIL- qHMS7 , both in the DJY1 background and investigated pollen fertility in the F 1 plant. We observed ~75% pollen sterility, being 50% earlier abortion (at the uninucleate stage, associated with the DJY1 allele of qHMS1 ) and 25% later abortion (at the binucleate stage, associated with the Mer allele of qHMS7 ), indicating that half of the 50% alive pollens (carrying the Mer allele of qHMS1 ) were later killed by the DJY1 toxin-antidote system of qHMS7 (Fig. 6a–e ). Consequently, nearly all the F 2 progeny contain at least one functional copy of the two toxin-antidote systems, thus verifying selective transmission of the pollen carrying both the Mer allele of qHMS1 and the DJY1 allele of qHMS7 (Fig. 6f–g ). Since only one genotype pollen ( 1 M/7D , denoting qHMS1-Mer/qHMS7-DJY1 ) in the F 1 plants heterozygous at both qHMS1 and qHMS7 is viable, four genotypes ( 1D1M/7D7M , 1 M1M/7D7M , 1D1M/7D7D and 1M1M/7D7D ) are expected at a 1:1:1:1 ratio in the F 2 population if the four female gametes ( 1D/7M , 1M/7M , 1D/7D and 1M/7D ) are transmitted equally (Fig. 6f ). However, we observed the highest frequency of the 1M1M/7D7D genotype and the lowest frequency of the 1D1M/7D7M genotype, biased from the expected equal segregation (Fig. 6g ). This result implies higher transmission rate of the female 1 M/7D gamete, suggesting that qHMS1 and qHMS7 together can lead to partial female gamete sterility although they each alone does not do so. Those results demonstrate that the two toxin-antidote systems are independent of each other in action and together can confer tiered reproductive isolation. Fig. 6: qHMS1 and qHMS7 are independent in action and together provide tiered hybrid male sterility. a – d Chromosome location of qHMS1 and qHMS7 and representative images of pollen phenotype in DJY1 ( a ), DJY1/ qHMS1 F 1 (F 1 -HMS1) ( b ), DJY1/ qHMS7 F 1 (F 1 -HMS7) ( c ) and qHMS1 / qHMS7 F 1 (F 1 -HMS1/7) ( d ). The pollen abortion caused by qHMS1 at uninucleate stage and that caused by qHMS7 at binucleate stage are indicated by pink arrowheads and black arrows, respectively. Scale bar, 100 μm. e Quantification of pollen phenotypes in hybrid plants. Data are means ± SD ( n = 5 independent spikelets). f Expected genotypes among progeny of F 1 -HMS1/7. Pink arrowheads indicate the aborted pollen. 1D , DJY1 allele of qHMS1 ; 1 M , Mer allele of qHMS1 ; 7D , DJY1 allele of qHMS7 ; 7 M , Mer allele of qHMS7 . g Genotypic distribution among progeny of F 1 -HMS1/7 plants ( n = 4 F 2 populations from four randomly chosen F 1 plants). The prevalence of the four genotypes verifies the expectation in f . Note the uneven distribution frequency of the four genotypes. The female gametes carrying both the functional TAs (1 M/7D) have the highest transmission whereas those carrying both the none-functional TAs (1D/7 M) have the lowest transmission, suggesting that two TAs together can build up partial hybrid female sterility. Four F 2 populations (100–200 plants each) from 4 randomly chosen F 1 plants were genotyped. Data are means ± SD. Source data are provided as a Source Data file. Full size image Understanding the genetic mechanism of hybrid male sterility in rice is not only a central issue in evolution biology, but also has directly important applications in breeding. Most of the causal genes responsible for hybrid male or female sterility were identified in the studies aimed to utilization of robust heterosis between subspecies of cultivated rice. Knocking out of some of those genes in either male or female parent has been recently shown to restore hybrid fertility to almost a practical level in seed production [41] . Wild rice species constitute important gene pools that can be exploited to develop new rice varieties with resistance to biotic and abiotic stresses and to challenge global climate changes. Cloning of genes governing hybrid sterility between wild and cultivated rice, followed by targeted mutagenesis to those genes may allow efficient gene flow from wild gene pools to modern cultivars. However, few studies have been focused on interspecific reproductive isolation. We started to work on hybrid male sterility between Mer (the most distant wild species in the AA genome group) and cultivated rice over a decade ago. In this study, we have identified causal genes at qHMS1 , as an addition to qHMS7 cloned previously [31] , thus moving one more step towards cloning of all the four mapped loci. Toxin-antidote systems are common in nature although the involved genes and encoded proteins are diverse among them. For example, the toxin-antidote element was first described as a single locus in the beetle Tribolium [42] . Cloning of the genes peel-1 and zeel-1 , encoding a naturally occurring sperm-derived toxin (a four-pass transmembrane protein) and antidote (a six-pass transmembrane protein), respectively, was reported in nematodes more than a decade ago [16] , [17] . Along with the discovery of more toxin-antidote systems in C. elegans [18] and C. tropicalis [43] , analogous effects between them were found, in which those elements act independently and when combined together, confer extensive genetic incompatibility. Although only a few have been reported in plants, including the one recently described in Arabidopsis [25] , the selfish genetic elements seem common in nature and likely play key role in speciation and maintenance of species identity. Different from those found in some other species, where a single gene can encode both toxin and antidote proteins, such as the wtf genes in saccharomyces pombe [14] , [15] , the Sk-1 genes in neurospora [24] and the Spok and Het-s genes in Podospora anserina [22] , [23] , plant selfish genetic elements are usually encoded by at least two genes. Interestingly, both the toxin-antidote systems at qHMS1 and qHMS7 are encoded by two linked genes. Whether this is specific to hybrid between Mer and O. sativa remains to be investigated in future studies. The proteins encoded by qHMS1 are completely different from those by qHMS7 . HPT and HPA belong to DEAD-like RNA helicases and F-box protein, respectively, whereas the toxin and antidote encoded by qHMS7 are RIP domain-containing protein and grass family-specific protein [31] , respectively. In addition, they also have different subcellular localizations (HPT in cytoplasm and nucleus and HPA in nucleus vs ORF2 in cytoplasm and nucleus and ORF3 in mitochondria). Regards of the timeline for pollen abortion, it is likely that qHMS1 exerts its effects prior to the action of qHMS7 . It is unknown if the protein features and localizations determine their action order. Moreover, the malfunctionization of qHMS1 in the latest species has clear simple path and more recent. In contrast, the evolution trajectory of functionization of qHMS7 is a long path and much more complicated [31] . However, we cannot exclude the possibility that the formation of functional qHMS1 had a long evolution trajectory before Mer . The DEAD-box helicases are a large family of conserved RNA-binding proteins that belong to the broader group of cellular DExD/H helicases and perform diverse cellular functions in virtually all steps of RNA metabolism from bacteria to humans [44] , [45] , [46] . F-box proteins function as substrate adaptors for the SCF ubiquitin ligase complexes, which mediate the proteasomal degradation of a diverse range of regulatory proteins [47] . The F-box protein-involved self-incompatibility/compatibility has been reported [48] , [49] , [50] , [51] . We hypothesize that HPT interferes RNA metabolisms related to early pollen development and HPA detoxifies HPT possibly through SKP1-CULLIN1-F-box (SCF)-mediated protein degradation. However, our in vitro assays did not detect their physical interaction, implying that the HPA-associated SCF complex may work on a substrate that in turn regulates HPT. On the other hand, HPT is synthesized in the cytoplasm and may be transported to the nucleus (in consistence with its subcellular localization), where it interferes with RNA metabolism. When nucleus-localized HPA is available, the HPT degradation process is triggered on, thus protecting pollens from abortion. HPT acts in a sporophytic manner whereas HPA in a gametophytic manner. It is possible that the cytoplasm-localized HPT (possibly shuttling in and out of nucleus) but not the nucleus-localized HPA in the pollen mother cell is transmitted through meiosis to the microspore, such that pollens lacking HPA fail to develop due to the presence of the toxin HPT. A recent study in maize establishes that gametophyte genome activation occurs at pollen mitosis I [52] . We therefore also postulate that the HPT transcript transcribed in the pollen mother cell may be more stable relative to that of HPA , survive meiosis until the microspore uninucleate stage and then be translated, killing pollens without HPA, as pollen abortion starts to be seen at the uninucleate stage (Supplementary Figs. 4 , 5 ). Why HPT is selectively toxic to male gametophyte, as also seen in other toxin-antidote systems [31] , [32] , remains mysterious. Nevertheless, we have decoded another quantitative locus, in addition to qHMS7 , in our endeavor to understand hybrid sterility control between the earliest wild rice and cultivated rice in the AA genome group. As approaching to clone other the two mapped loci [31] , we expect that knocking out multiple hybrid sterility genes would provide interesting insight into breaking reproductive isolation formed during million years evolution, to finally realize more efficient gene flow from wild to cultivated rice. Plant material and growth condition The wild rice Oryza meridionalis (accession 104498, Mer ) and the O. sativa ssp. japonica cultivar Dianjingyou1 (DJY1) were used to produce F 1 . The F 1 plant was then backcrossed for 5 times using DJY1 as the recurrent parent and the resulting BC 5 F 1 was self-pollinated to finally generate the near-isogenic line NIL- qHMS1 . Genetic background of NIL- qHMS1 was scanned using 453 simple sequence repeat (SSR) markers evenly distributed on the 12 chromosomes (Supplementary Fig. 1 and Supplementary Data 3 ). All the wild rice and cultivated rice species used for evolutionary analysis were either maintained in our lab or provided by the Chinese Crop Germplasm Resources Center (Beijing, China). All plants were grown in field at our experimental stations in Nanjing or Beijing during the summer season, or in Sanya, South China during winter season. Evaluation of pollen fertility Spikelets collected from plants at the flowering stage were fixed in Carnoy’s fixative (100% ethanol: 100% acetic acid = 3:1). Pollen grains from the fixed spikelets were stained by 1% (w/v) iodine-potassium iodide (I 2 -KI) solution. At least three spikelets (~ 200 pollens counted each) were examined for pollen fertility under a light microscope (Leica DM5000 B). Dark-stained pollen grains were scored as fertile, whereas irregular-shaped, unstained grains were scored as sterile. Pollen fertility is measured by Image J software. Cytological analyses The developmental course of anthers was classified into 14 stages [53] , [54] . For semi-thin sections, anthers of different developmental stages were first fixed in Carnoy’s fixative, underwent a series of ethanol dehydration and resin penetration, and then were embedded in resin (Technovit 7100, Hereaus Kulzer). Sections were prepared using an EM UC7 Ultramicrotome (Leica), adhered to a glass slide, and then stained with 0.25% toluidine blue O (Chroma Gesellshaft Shaud). Images were captured using a light microscope (Leica DM5000 B). For aceto-carmine staining, the microspores were released onto the slide by breaking anthers fixed in Carnoy’s fixative and stained with 1% (w/v) aceto-carmine solution. two minutes later, the samples were examined under a light microscope. The observation was repeated 3 times (one spikelet per replicate) for each developmental stage to calculate the frequency of microspores (or pollen grains) of different types. The procedure of DAPI (4’, 6-diamidino-2-phenylindole) staining was basically the same as for the aceto-carmine staining, except that the dye was replaced with DAPI and glycerin. The samples were examined under a fluorescence microscope (Leica DM5000 B). For SEM and TEM analysis, spikelets at the mature stage were fixed in 2.5% (v/v) glutaraldehyde for 24 h to 72 h, post-fixed by 1% OsO 4 in PBS, pH 7.2. After dehydrating through an ethanol series, samples were placed in Spurr’s resin and then ultrathin sectioned. Furthermore, sections were double-stained with 2% (w/v) uranyl acetate and 2.6% (w/v) lead citrate aqueous solution, and examined with a Jeol 100 CX electron microscope (Jeol Ltd, Tokyo, Japan). Fine mapping of the qHMS1 locus The qHMS1 locus was first delimited to a genomic interval between the markers CH1-11 and RM3475 using 356 BC 5 F 2 and 8 molecular markers. A series of Indel markers were designed based on genomic sequence difference nearby the mapped region between Oryza meridionalis and Nipponbare ( O. sativa, japonica ) at the Gramene website ( http://www.gramene.org/ ). The SNP markers were based on sequences of site-specific PCR products amplified from DJY1 and NIL- qHMS1 , respectively. For fine mapping, 11,800 plants from the progeny of the BC 5 F 2 population were screened for recombinants using the two Indel makers (E1-3 and E1-6). Finally, the qHMS1 locus was delimited to a 43-kb genomic region between the SNP markers C1-20 and C1-39. All the primers for mapping are listed in Supplementary Data 4 . RNA isolation and quantitative reverse transcription PCR analysis Various tissues at the flowering stage and anthers at defined development stages were collected from DJY1, NIL- qHMS1 and F 1 plants and stored at −80 °C. Total RNA was extracted using an RNA Prep Pure Plant Kit (TIANGEN). The first strand cDNA was synthesized using Prime Scriptase (TaKaRa). Quantitative real-time RT-PCR, with 3 biological replicates, was performed using SYBR Premix Ex Taq II (TaKaRa) on an Applied Biosystems 7500 Real-Time PCR System. Amplifications were performed at 95 °C for 5 s, 60 °C for 34 s, 40 cycles. The UBQUITIN1 ( LOC_Os03g13170 ) gene was used as an internal control. All the primers used in this analysis are listed in Supplementary Data 4 . RNA-Sequence analysis The spikelets of DJY1, NIL- qHMS1, and F 1 were collected at stages 9 to 11 and the anthers of gHPT-COM and DJY1 were collected at the meiotic stage and the uninucleate stage. Total RNA of different tissues was extracted according to the above method and RNA-Sequencing libraries were prepared with three biological replicates. Then, the libraries were sequenced separately using Illunima HiSeq X-10 platform (Biomarker Biotechnology Co) and generated reads were cleaned and then mapped to the Nipponbare reference genome using the HISAT [55] and Bowtie2 [56] tools. RNA-Sequence data was browsed using IGV software. CRISPR/Cas9 vector construction The 20-bp target-specific spacer sequences were synthesized, fused with the AarI linearized intermediate vector SK-Grna and introduced into CRISPR-Cas9 binary vector pCAMBIA1305 to generate knock-out constructs [57] . Then, these vectors were transformed into the callus of DJY1, NIL- qHMS1 or F 1 via an Agrobacterium tumefaciens–mediated transformation system [58] . Transgenic plants were regenerated from transformed callus by selection on hygromycin-containing medium. The edited types of transformants were identified by sequencing. Genes sequences were analyzed using Geneious software. Primers used in the plasmid construction are listed in Supplementary Data 4 . Genetic complementation The full-length genomic fragments of corresponding genes were obtained from DJY1 and NIL- qHMS1 by PCR amplification. Then, these fragments were fused into the vector pCUbi1390 using the In-Fusion Advantage PCR Cloning Kit (Clontech) to generate 1390- HPT- D, 1390- HPT- M, and 1390- HPA-M genetic complementation vectors. These vectors were transformed into the callus of DJY1, NIL- qHMS1 or F 1 via an Agrobacterium mediated transformation system. Positive transgenic individuals were identified through PCR using transgene-specific primers. All primers used for plasmid construction are listed in Supplementary Data 4 . Subcellular localization The full-length CDSs of HPT and HPA without stop codons were fused with a green fluorescent protein (GFP) and inserted into the pAN580-GFP vector to produce pAN590-3-D-GFP, pAN590-3-M-GFP and pAN590-5-M-GFP constructs. Rice protoplasts was prepared as the following steps: the stems of 9311 seedlings, which had been growing for 7–10 days, were cut into small segments of about 1–2 mm and placed in 10 ml of 0.6 M mannitol for 10 min. Remove mannitol, add 10 ml enzyme solution (activated at 42 °C), shake at 25 °C at 60 rpm, enzymatic hydrolysis for 5 h. Remove the enzyme solution, add 30 ml W5 solution in two batches, shake gently, pass through a 200-mesh sieve, and collect the filtrate. Centrifuge at 1000 rpm for 3 min and remove the supernatant. Rinse with 4 ml W5 solution once, centrifuge and remove supernatant. The protoplasts were obtained by adding 2 ml MMG solution for re-suspension [59] . Plasmid DNA of sequence-confirmed pAN580-GFP and the nuclear marker D53-mCherry (as control) were co-transformed into rice protoplasts and incubated in darkness for 16 h at room temperature. Subcellular distribution of GFP fluorescence was visualized using a confocal laser scanning microscope (Zeiss LSM 780). All the primers used here are listed in Supplementary Data 4 . Transactivation assays An approximately 2.5-kb promoter region of HPT-D and HPT-M , 2.7-kb promoter region of HPA-D and 1.6-kb promoter region of HPA-M were amplified from DJY1 or NIL- qHMS1 genomic DNA by PCR and cloned into the pGreenII0800-LUC vector to generate P- HPT-D , P- HPT-M , P- HPA-D and P- HPA-M LUC reporter constructs. Sequencing confirmed plasmids DNA were transformed into rice protoplasts [59] . The luciferase gene from Renilla reniformis (Ren) under control of the CaMV35S promoter was used as the internal control. The LUC activity was calculated with a Dual-Luciferase Assay Kit (Promega E2920) following the manufacturer’s recommendations using the TriStar2 Multimode Reader LB942 (Berthold Technologies) and the relative LUC activity was represented by the ratio of LUC/Ren. All the primers used here are listed in Supplementary Data 4 . β-Glucuronidase (GUS) histochemical staining An approximately 1.6-kb promoter fragment upstream of the start codon of HPA-M were amplified from NIL- qHMS1 genomic DNA by PCR and cloned into the binary vector pCAMBIA1381 to drive GUS reporter gene expression. Then, this vector was transformed into the callus of NIL- qHMS1 via an Agrobacterium tumefaciens–mediated transformation system. Young spikelets from positive T 0 plants were stained with GUS dye and decolorized with 75% alcohol [60] . Images were captured using a light microscope (Leica DM5000 B). The primers for PCR amplification are listed in Supplementary Data 4 . Yeast two-hybrid (Y2H) assays Y2H assays were performed using the Matchmaker Two-Hybrid System (Clontech, CA, USA) following the manufacturer’s protocol. The coding sequence of HPA was amplified and cloned into the pGBKT7 vector (bait), while the HPT was cloned into the pGADT7 vector (prey). These two constructs were co-transformed into yeast strain AH109 and selected on medium plates without Leu and Trp (SD/-Leu-Trp) at 30 °C for 3–5 days. The interactions were tested on selective medium (SD/-Leu-Trp-His) and (SD/-Leu-Trp-His-Ade) plates. Primers used in the assays are listed in Supplementary Data 4 . Protein pull-down assay The coding sequence of HPA was introduced into the pMAL-C2x vector to construct the fusion protein MBP-HPA, and HPT was cloned into the pGEX-4T-2 vector to make the GST-HPT fusion protein (primers used in the assays are listed in Supplementary Data 4 ). The proteins including fusions and empty tags were expressed in Escherichia coli DE3 cells (TransGen). Different combinations of proteins expressed in vitro were mixed together and incubated with GST-beads overnight [61] . The pull-down assays were performed and samples were detected with anti-GST direct antibody (WBL) or anti-maltose-binding protein (anti-MBP) (NEB) monoclonal antibody at 1: 5000 dilution, and the secondary antibody was anti-IgG (WBL) mouse (1: 5000 dilution; Abmart). The ECL reagent (Bio-Rad) was used to test the immunoblot. RNA in situ hybridization Young spikelets from DJY1 and NIL- qHMS1 were fixed in a FAA (RNase free) fixative solution at 4°C. Through dehydration in a series of ethanol and xylene, simples were embedded in paraffin (Paraplast Plus, Sigma). A probe was prepared by amplifying a fragment from HPA-M cDNA and cloned into the pGEMT Easy vector (Promega). The probe was then transcribed in vitro using a DIG Northern Starker Kit (Cat. no. 2039672, Roche) following the manufacturer’s instructions. RNA in situ hybridization with the probes were performed on transverse sections of anther. After blotting with Antidigoxigenin AP-conjugated (Roche, 11093274910) and incubation with the NBT solution (Roche, 11383213001), the slides were observed and photographed using a light microscope (Leica DM5000 B) [60] . Primers used are listed in Supplementary Data 4 . Amino acid sequence alignment The full-length amino acid sequence of HPT and HPA were used to search the homologous sequences in the National Center for Biotechnology Information (NCBI, http://www.ncbi.nlm.nih.gov/ ). Amino acid sequence alignment was constructed using Bioedit software. Phylogenetic tree was constructed using MEGA-X software (neighbor-joining method with 1000 bootstrap replicates). Reporting summary Further information on research design is available in the Nature Portfolio Reporting Summary linked to this article.